Lateral pH gradient between OXPHOS complex IV and F0F1ATP-synthase in folded mitochondrial membranes Ion-driven ATP synthesis by rotary F 0 F 1 ATP-synthase powers aerobic life. Since Mitchell’s seminal hypothesis, this synthesis has been discussed in terms of the proton-motive force between two bulk phases, each in equilibrium. In active mitochondria, a steady proton flow cycles between pumps and the distant ATP synthase. Here we determine the lateral pH profile along the p-side of cristae in situ by attaching a ratiometric fluorescent pH-sensitive GFP variant to OXPHOS complex IV, a proton pump, and the dimeric F 0 F 1 ATP-synthase, a proton consumer. In respiring HeLa cells, we observe that the local pH at F 0 F 1 dimers is 0.3 units less acidic than that at complex IV. This finding is consistent with the calculated pH profile for steady proton diffusion from CIV to F 0 F 1 . The observed lateral variation in the proton-motive force necessitates a modification to Peter Mitchell’s chemiosmotic proposal. The experimental technique can be extended to other pH-dependent reactions in membrane microcompartments. In eukaryotic cells, adenosine triphosphate (ATP) is produced at the crista membrane of mitochondria. Cristae are flat invaginations of the mitochondrial inner membrane that extrude into the matrix space with a few tubular openings to the inter-membrane space between the inner and outer membranes [1] , [2] , [3] . The crista membrane hosts the components of the respiratory electron transport chain (complexes I-IV, alias CI-IV) and ATP synthase (complex V, F O F 1 alias CV). Complexes I, III and IV pump protons from the matrix (the n-side of the membrane) into the intra-cristae space (the p-side). The proton-motive force drives protons back via ATP synthase and ATP is formed [4] , [5] . The proton pumps and the proton-driven ATP synthase can be segregated. Complexes I-IV are mainly found in the flat sheet membrane [6] , [7] , whereas immuno-EM and EM-tomography have revealed ribbons of F 0 F 1 dimers lining the highly curved rim [8] , [9] , [10] , [11] , [12] . These ribbons seem to be involved in folding the crista membrane. Deleting certain subunits of F 0 F 1 (termed e and g) abolishes the dimerization, and thus the high curvature of the crista membrane without deactivating ATP synthesis [13] . The accumulation of ATP synthase in the highly curved rim has recently introduced a new dimension to the classical debate over localised versus delocalized (that is, chemiosmotic) proton coupling: electrostatic guidance of protons into ATP synthase. One group has postulated that the curved membrane segment concentrates protons at the concave side of the membrane, thereby generating extra proton-motive force for ATP synthesis in cristae [9] . A related process for the thylakoid membranes of chloroplasts has been coined ‘Proton-Electrostatic Hypothesis for Localized Proton Coupling Bioenergetics’ [14] . Both proposals are based on the electrostatics at low ionic strength where protons and hydroxyl anions were the major charge carriers. In contrast, for a realistic situation (physiological ionic strength and steady proton flow), we expect the local pH at the p-side of CV (the proton sink) to be more alkaline and not more acidic than the pH at CIV (the proton source). Here, this expectation is tested using a pH-indicating analogue of green fluorescent protein. This analogue is fused to the p-side (intermembrane/intra-cristae space) of either CIV or dimeric CV. The local pH at either CIV or the CV dimer is measured in actively respiring mitochondria of HeLa cells. To intensify OXPHOS, the cells are cultured in galactose plus glutamine [15] to circumvent ATP production by glycolysis. In contrast to hyperglycaemic conditions, these metabolic substrates force HeLa cells to rely on OXPHOS and CV-dimer stabilisation [16] . These conditions result in a lateral pH difference between CIV and the dimeric synthase in the intra-cristae space: the determined proton concentration at the ATP synthase molecules in the dimer ribbons around the perimeter of cristae differs from the concentration predicted by the previously described electrostatic approaches. The following treatment of diffusive proton flow under physiological conditions provides an explanation for this difference. Local pH determination at specific OXPHOS complexes To measure local pH values, superecliptic pHluorin (sEcGFP) fused to subunits of OXPHOS complexes IV and V was used as a local pH indicator [17] . SEcGFP is a double emission fluorescent protein. OXPHOS subunits were tagged at their C terminus and checked for correct localisation in mitochondria. SEcGFP was excited with a 405-nm laser, and the fluorescence emission was recorded simultaneously at 454–474 nm and 508–514 nm. The local pH was inferred from the emission ratio (Em 511/464 ) [18] . In one transiently transfected HeLa cell line, sEcGFP was fused to the C terminus of subunit 8a of CIV, which is located at the p-side (PDB ID: 2EIN). In the second cell line, sEcGFP was fused to the dimer-specific subunit e of CV, which is also located at the p-side in the rims of cristae [19] . The tagging of these subunits did not interfere with their localisation inside mitochondria ( Fig. 1a,b ), and no indication of functional impairment was found from oxygen consumption recording [20] and membrane potential measurements ( Fig. 1c ). The emission ratio images were intrinsically different ( Fig. 1a,b ). Calibration was performed with sEcGFP tagged to the proteins of interest in the respective cell lines under conditions in which the membranes were permeable to protons. The buffer pH was adjusted, and the resulting fluorescence emission ratio was recorded ( Fig. 1d ). 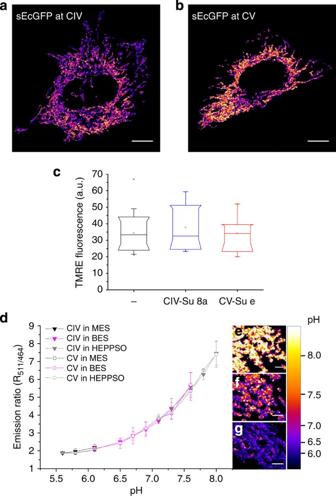Figure 1: Calibration of the pH indicator sEcGFP at functional subunits of OXPHOS complexes in the intra-cristae space. (a,b) Fluoro-micrographs of HeLa cells with sEcGFP at subunit 8a of CIV (a) and subunit e of CV (b) show the mitochondrial localisation of the tagged subunits. (c) The labelling of subunits 8a (CIV) and Su e (CV) with the pH indicator sEcGFP does not influence the functionality, as indicated by the membrane potential ΔΨmmeasurements. The relative TMRE fluorescence in HeLa cells, CIV-sEcGFP- and CV-sEcGFP-expressing cells was determined as a measure of the membrane potential ΔΨmin the presence of 5 nM TMRE. Statistics: (n=2 independent transfections with >15 cells each). The boxes represent the 10th to 90th percentiles with the 25th to 75th percentiles within the narrower part of the box. The vertical lines in the boxes represent the median values. The square symbols in the boxes denote the respective mean values. The error bars denote the 5th to 95th percentile values. The minimum and maximum values are denoted by x. (d) Ratiometric response of SEcGFP to the local pH. CCCP, nigericin and oligomycin were used to equilibrate the cell to the pH of the buffer. The fluorescence ratios at pH 6.1, 7.1, 7.3 and 7.6 pH were determined in two different standard buffers. Every data point representsn=2 independent experiments and mean values±s.d. from at least 10 cells. (e–g) The ratiometric pH values in mitochondria were colour coded according to the look-up table on the right. Scale bars: 10 μm (a,b), 2 μm (e–g). Figure 1: Calibration of the pH indicator sEcGFP at functional subunits of OXPHOS complexes in the intra-cristae space. ( a , b ) Fluoro-micrographs of HeLa cells with sEcGFP at subunit 8a of CIV ( a ) and subunit e of CV ( b ) show the mitochondrial localisation of the tagged subunits. ( c ) The labelling of subunits 8a (CIV) and Su e (CV) with the pH indicator sEcGFP does not influence the functionality, as indicated by the membrane potential ΔΨ m measurements. The relative TMRE fluorescence in HeLa cells, CIV-sEcGFP- and CV-sEcGFP-expressing cells was determined as a measure of the membrane potential ΔΨ m in the presence of 5 nM TMRE. Statistics: ( n =2 independent transfections with >15 cells each). The boxes represent the 10th to 90th percentiles with the 25th to 75th percentiles within the narrower part of the box. The vertical lines in the boxes represent the median values. The square symbols in the boxes denote the respective mean values. The error bars denote the 5th to 95th percentile values. The minimum and maximum values are denoted by x. ( d ) Ratiometric response of SEcGFP to the local pH. CCCP, nigericin and oligomycin were used to equilibrate the cell to the pH of the buffer. The fluorescence ratios at pH 6.1, 7.1, 7.3 and 7.6 pH were determined in two different standard buffers. Every data point represents n =2 independent experiments and mean values±s.d. from at least 10 cells. ( e – g ) The ratiometric pH values in mitochondria were colour coded according to the look-up table on the right. Scale bars: 10 μm ( a , b ), 2 μm ( e – g ). Full size image The resulting pH titration curves were congruent, independently of the location of attachment of the pH indicator and independently of the chemical nature of the buffer. For pH determination, a mean titration curve was used. The fluorescence emission ratio was correlated with the pH, and the ratio images of the mitochondria were accordingly colour coded ( Fig. 1e–g ). Local pH in respiring cristae is higher at CV than at CIV We next checked the local pH at a cytochrome c oxidase proton pump in the intra-cristae space. SEcGFP was fused to subunit 8a in CIV and faced the intra-cristae space. CIV is mainly found in the sheet region of cristae [6] , [7] . Concurrently, the local pH at F 0 F 1 ATP-synthase, which pumps protons back into the matrix under ATP synthesising conditions, was determined. SEcGFP was fused to subunit e in CV. Subunit e is involved in the dimerisation of CV [21] and is also localised in the intermembrane space, mostly at the rims of cristae [22] . 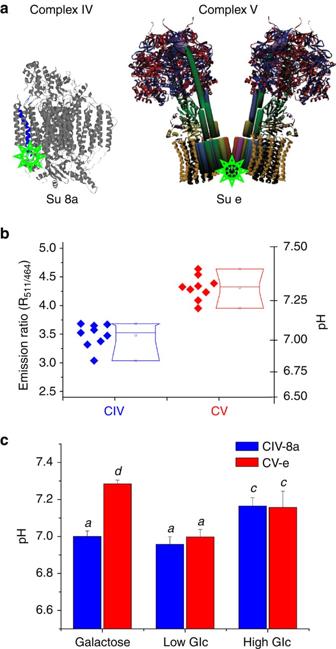Figure 2: Local pH values at CIV and FOF1ATP-synthase in actively respiring HeLa mitochondria. (a) Structural models of complex IV and the CV dimer attached to sEcGFP (green). (b) Box-and-whisker plot and mean data points (each data point represents the mean of 5 cells in one experiment) showing the fluorescence emission ratio (left scale) and the corresponding local pH (right scale) at the proton pump (CIV) and at F0F1synthase (CV) in the intra-cristae space of transiently transfected cells. The boxes represent the 10th to 90th percentiles with the 25th to 75th percentiles within the narrower part of the box. The vertical lines in the boxes represent the median values. The square symbols in the boxes denote the respective mean values. The error bars denote the 1st and 99th percentile values. The minimum and maximum values are denoted by x. The local pH was inferred from the emission ratio using the mean titration curve fromFig. 1. (c) Mean pH values at CIV and CV under various nutrition conditions (mean±s.e.m.; significance levels determined by a one-way ANOVA (a,b):P⩽0.05; (a–c):P⩽0.01; (a–d):P⩽0.001;n=9 independent experiments with 45 determined values for respiration and low glucose;n=2 independent measurements and 14 data points for high glucose). Media: respiration with glutamine (2 mM) and galactose (10 mM); glycolysis with a low (5.5 mM) and high glucose (25 mM) supply. Figure 2 illustrates the molecular localisation of the pH indicator (sEcGFP) fused to subunit 8a (Su 8a) in CIV and subunit e (Su e) in (CV) 2 ( Fig. 2a ). Fluorescence emission ratios were recorded for sEcGFP-CIV (Su 8a) and sEcGFP-CV (Su e). The obtained fluorescence emission ratios of the location-specific sensor clearly indicate a higher proton concentration at CIV (lower pH) and a lower concentration at the CV dimers (higher pH) ( Fig. 2b ). These data show that the local pH at the proton pump (CIV) was 0.3 units more acidic than that at the proton sink (CV). We attribute this difference to the respective proton pumping and consuming activities at the different positions of the folded cristae membrane. This difference was obtained for actively respiring mitochondria supplied with galactose. Figure 2: Local pH values at CIV and F O F 1 ATP-synthase in actively respiring HeLa mitochondria. ( a ) Structural models of complex IV and the CV dimer attached to sEcGFP (green). ( b ) Box-and-whisker plot and mean data points (each data point represents the mean of 5 cells in one experiment) showing the fluorescence emission ratio (left scale) and the corresponding local pH (right scale) at the proton pump (CIV) and at F 0 F 1 synthase (CV) in the intra-cristae space of transiently transfected cells. The boxes represent the 10th to 90th percentiles with the 25th to 75th percentiles within the narrower part of the box. The vertical lines in the boxes represent the median values. The square symbols in the boxes denote the respective mean values. The error bars denote the 1st and 99th percentile values. The minimum and maximum values are denoted by x. The local pH was inferred from the emission ratio using the mean titration curve from Fig. 1 . ( c ) Mean pH values at CIV and CV under various nutrition conditions (mean±s.e.m. ; significance levels determined by a one-way ANOVA ( a , b ): P ⩽ 0.05; ( a – c ): P ⩽ 0.01; ( a – d ): P ⩽ 0.001; n =9 independent experiments with 45 determined values for respiration and low glucose; n =2 independent measurements and 14 data points for high glucose). Media: respiration with glutamine (2 mM) and galactose (10 mM); glycolysis with a low (5.5 mM) and high glucose (25 mM) supply. Full size image Next, we compared different nutrition conditions. It is known that the type of energy substrate modulates the mitochondrial oxidative capacity and respiration in cancer cells, such as HeLa cells [15] , [23] . With low glucose, the intra-cristae space was acidified, and no difference was measured between CIV and CV. Reverse ATP synthase has been suggested to maintain Δμ H + by pumping protons out of the matrix when respiratory proton pumping is insufficient [24] . The sink will then become a source. Our data are consistent with this interpretation. Supplementing cells with high glucose (4.5 g l −1 ) also abrogated the difference in the lateral pH between the source and sink, but the pH generally increased ( Fig. 2c ). In these conditions, cells gain ATP mostly by substrate chain phosphorylation in glycolysis, and both respiration [16] , [23] and proton pumping are reduced. In addition, hyperglycaemia obviously is accompanied by a decrease in the number of F 0 F 1 ATP-synthase dimers [16] . Inhibitors and protonophores eliminate the lateral pH gradient We also tested the significance of the lateral pH difference in respiring cells by using inhibitors and protonophores. The difference was expected to disappear when the membrane was permeable to protons (by the addition of the protonophore CCCP in this study) or when the proton cycling was blocked at F 0 F 1 ATP-synthase (by the addition of oligomycin in this study). The cell structure was not obviously altered upon the addition of either CCCP or oligomycin ( Fig. 3a,b ) within the first 50 min. Both agents equilibrated the local pH values at CIV and CV, as projected. The pH values shifted into acidity (by oligomycin, especially after 30–50 min) and towards a medium pH (by CCCP), also as expected ( Fig. 3c ). Total equilibration with the medium pH was only observed after prolonged CCCP treatment, which led to mitochondrial fragmentation in some cells and changes in cell shape. The induced acidification of the intermembrane space after prolonged oligomycin treatment is expected because F 0 F 1 ATP-synthase (the sink) is blocked by oligomycin while the proton pumps (source) of the galactose-grown cells still function. These pH changes will continue until a feedback mechanism stops them. In comparison with the CCCP treatment, the inhibition of CIV by KCN caused an even stronger pH increase in the intra-cristae space, as expected if the proton pumping activity of this terminal oxidase was effectively blocked. KCN led to rapid mitochondrial fragmentation and cell shape changes ( Fig. 3d ), which are unwanted side effects. The pH results provide further evidence in favour of the localisation of the pH sensor at the p-side of the membrane. 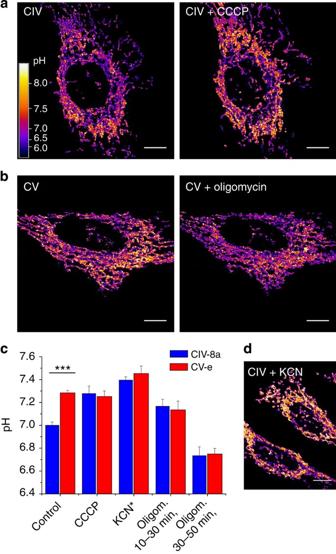Figure 3: Protonophore and inhibitor effects on the local pH values in the intra-cristae space. Effects of short circuiting ((a), 10 μM CCCP) and blocking ((b), 5 μg ml−1oligomycin) of the cyclic flow of protons between CIV and CV. (c) Ratiometrically determined local pH under the above mentioned conditions compared with that in untreated cells (control). The pH of the medium was 7.5. CCCP (10 μM):n=4 independent experiments and 20 cells; KCN (3 mM):n=1 experiment and 7 cells; 10–30 min oligomycin: n=4 independent experiments and 20 cells; 30–50 min oligomycin:n=4 independent experiments and 20 cells. *Because of the rapid fragmentation of KCN-treated mitochondria, these measurements were not pursued. Mean±s.e.m.; significance levels were determined between the CIV values and the CV values for each treatment using a one-way ANOVA ***P⩽0.001 (d) Fluoro-micrograph showing fragmented mitochondria after KCN treatment (3 mM, 10 min) in CIV-Su8a-sEcGFP-transfected cells. Scale bars, 10 μm. Figure 3: Protonophore and inhibitor effects on the local pH values in the intra-cristae space. Effects of short circuiting (( a ), 10 μM CCCP) and blocking (( b ), 5 μg ml −1 oligomycin) of the cyclic flow of protons between CIV and CV. ( c ) Ratiometrically determined local pH under the above mentioned conditions compared with that in untreated cells (control). The pH of the medium was 7.5. CCCP (10 μM): n =4 independent experiments and 20 cells; KCN (3 mM): n =1 experiment and 7 cells; 10–30 min oligomycin: n=4 independent experiments and 20 cells; 30–50 min oligomycin: n =4 independent experiments and 20 cells. *Because of the rapid fragmentation of KCN-treated mitochondria, these measurements were not pursued. Mean±s.e.m. ; significance levels were determined between the CIV values and the CV values for each treatment using a one-way ANOVA *** P ⩽ 0.001 ( d ) Fluoro-micrograph showing fragmented mitochondria after KCN treatment (3 mM, 10 min) in CIV-Su8a-sEcGFP-transfected cells. Scale bars, 10 μm. Full size image Diffusion limitation counteracts the lateral pH equilibration When the proton pumping and consuming activities of the OXPHOS complexes are located at different positions in the flat crista membrane, the diffusion of protons becomes an important issue. The stationary proton diffusion between sources and sinks in a disk-shaped crista was simulated using the following simplifying assumptions, which are illustrated in Fig. 4 : 1 The intra-cristae space is a flat disk of radius R and thickness h . 2 Proton pumps are homogeneously distributed over the flat portions of the disk membrane. 3 Dimers of CV line the perimeter of the disk. 4 Cristae junctions are obstructed. 5 The total flux of protons into the ring of ATP synthase molecules, I tot ( R ) (mol × s −1 ), is constant due to the dominant role of the electric driving force. 6 Lateral proton flow between CIV and CV is diffusive without drift, due to the high ionic strength. 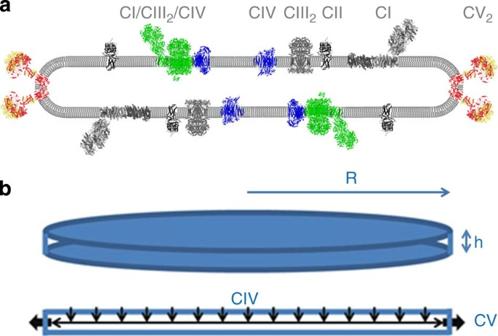Figure 4: Schematic representation of a crista with proton flow. (a) Cross section with proton pumps (CIV in blue as a monomer and in the supercomplex CI-CIII2-CIV) in the flat membrane and proton sinks (CV dimers, red) at the curved rim. (b) Overview and cross section with black arrows illustrating the proton flow (see text). Figure 4: Schematic representation of a crista with proton flow. ( a ) Cross section with proton pumps (CIV in blue as a monomer and in the supercomplex CI-CIII 2 -CIV) in the flat membrane and proton sinks (CV dimers, red) at the curved rim. ( b ) Overview and cross section with black arrows illustrating the proton flow (see text). Full size image The total flux at radius r , I tot ( r ) (mol s −1 ), depends on the diffusive flux density at this radius, J ( r ) (mol × m −2 × s −1 ), as follows: The total fluxes at the given radii r and R are proportional to the respective disk areas that are homogeneously filled with proton pumps such that and hence The diffusive flux density across any ring of radius r , , obeys Fick’s second law: where D (m 2 × s −1 ) is the diffusion coefficient of the protons. With equation (2), the solution of Fick’s equation becomes the following: Averaging over a homogenous distribution of CIV over the disk leads to the following solution: With the given assumptions, the calculated proton concentration drops parabolically from the centre of the disk-shaped membrane towards the ring of CV dimers at the perimeter. Using equation (5), we calculated the drop in the proton concentration from the centre to the perimeter of a crista ( R =0.5 μm) using a reasonable assumption for the total flux ( ), the thickness of the intra-crista space ( h =10 nm), and the diffusion coefficient of a proton ( ) in the crowded and diffusion-obstructed intra-crista space (see ref. 25 ). The calculated concentration drop was 80 nM from the centre of the crista disk (pH 6.8) to the perimeter. This drop is equivalent to a pH increase of 0.7 units from the centre (assumed pH 6.8) to the rim (calculated pH 7.5). The mean concentration drop was 40 nM (see equation (6)). The calculated values follow the same pattern as in the experiments; they are not meant to match quantitatively because the idealizations underlying the above solution do not strictly hold. ATP synthase molecules are not restricted to the perimeter at the rims of cristae [26] , the proton pumps may be non-homogeneously distributed over the flat surfaces, and the crista junction may not be perfectly proton tight. All these complications, however, do not invalidate the finding that the proton concentration at the inlet of the ATP synthase dimers is lower but not higher than the concentration elsewhere in the intra-cristae space. In the present study, we experimentally determined the lateral pH difference between the respiratory chain complex cytochrome c oxidase (proton pump) and F 0 F 1 ATP-synthase dimers (proton consumer). The two OXPHOS complexes are located at different positions in flat, hollow crista discs. CIV is mainly found in the sheet region [6] , [7] , while F 0 F 1 ATP-synthase dimers shape the rim [8] , [27] , [28] , [29] . Under respiratory conditions, the actual pH at the F 0 F 1 dimers at the rims of cristae was higher than the pH at the proton pump in the sheet region. Thus, the specific architecture of cristae with dimerisation and ribbon formation by ATP synthase does not enhance but rather diminishes the local proton-motive force for ATP synthesis. This result qualifies the contradictory claims of two other groups [9] , [14] . In his chemiosmotic hypothesis [4] , [5] , Peter Mitchell considered two bulk phases, and he assumed a constant proton-motive force across the coupling membrane. According to the data and the diffusion calculated in the present work, this assumption does not apply for a steady proton flow between a proton pump and a remote dimeric ATP synthase. For mitochondria, however, the amendment to Mitchell’s original concept is minor. While the entropic contribution to the proton-motive force (−2.3 RTΔpH) varies laterally, the electric component (FΔΨ) is not affected due to the high ionic strength. Slightly lowering the transmembrane pH difference at the ATP synthase dimers on the rim of cristae is intrinsically unfavourable to ATP production by CV dimers. By folding the cristae, however, dimerisation increases the packing density of the energy-transducing membrane and therewith the ATP production per volume. Some CV molecules reside in cristae sheets [7] , [26] . In hyperglycaemic conditions, which have been reported to decrease the number of CV dimers, the pH difference between CIV and CV disappears, as shown here. In addition, inhibitor effects eliminated the lateral difference between CIV and CV, as expected. Effective inhibition of the respiratory chain electron flow due to CIV inhibition by KCN also increased the intra-cristae space pH but was accompanied by unwanted ultrastructural changes and mitochondrial fragmentation. In contrast, during oligomycin treatment, acidification of the IMS proceeded due to the continuing activity of the proton pump. At the same time, the lateral pH gradient between CIV and CV vanished because of the inhibition of the sink, which switches the system from a steady state to equilibrium. In conclusion, the intra-cristae space obviously is a microcompartment with different structural and functional domains. Recently, 10–80 s pH pulses were found in the mitochondrial matrix [30] , [31] . The pulses should correspond to an alkalinisation of the intermembrane space. We cannot rule out the possibility that such pulses were recorded without being recognized. It is certainly challenging to address this possibility in the future. The observations in the present study ought to be of interest for ATP synthesis in all kingdoms of life. Chloroplasts have achieved even higher packing densities in their thylakoid membranes than found in cristae membranes. Despite its intricate folding, the thylakoid membrane forms a simply connected sheet in which the electric potential difference is delocalised over more than 10,000 ATP synthase molecules (see ref. 32 ); however, the pH difference may also vary laterally, as established for mitochondria in this work. In alkaliphilic bacteria, the close proximity of complex V to a proton pump may be essential for ATP synthesis to occur with virtually zero bulk-to-bulk proton-motive force (see refs 12 , 27 , 33 , 34 , 35 , 36 ). Plasmid constructs For eukaryotic expression, the full-length protein-coding region of superecliptic pHluorin (F64L/S65T/S147D/N149Q/V163A/S175G/S202F/Q204T/A206T) (a gift from Prof. Jürgen Klingauf) was inserted by PCR amplification into a modified pSEMS-26 m vector from NEB Biosciences (formerly Covalys Biosciences) using the following primers: forward 5′-GCGC GAATTC ACCATGAG TAAAGGAGAAGAACTTTTCACTGGAG-3′ and reverse 5′-GCGC GGATCC ACCGGTTTTGTATAGTTCATCCATGCCA TG-3′, with an Eco RI (forward) and a Bam HI (reverse) restriction site (underlined). The respective subunits of OXPHOS complexes were fused with their C termini to the N terminus of sEcGFP using the following primers: 5′-GCGC GATATC ATGTTGGCTACCAGGG-3′ (forward) and 5′-GCGC GAATTC CTTCTTCCACTCGTTCTTTTC G-3′ (reverse) for CIV-Su 8a, and 5′-GCGTAA GATATC ATGGTGCCACCGGTGCAGG-3′ (forward) and 5′-GCAATT GAATTC CTTTAATATGCTGTCATCTTCTG-3′ (reverse) for CV Su e (the EcoRV and EcoRI restriction sites are underlined) [20] . PCR primers were purchased from Sigma Aldrich. Enzymes, restriction buffer and BSA were purchased from NEB Biosciences. Cell culture and treatments HeLa cells, purchased from DSMZ (Deutsche Sammlung von Mikroorganismen und Zellkulturen GmbH), were cultured in minimal essential medium with Earle’s salts (MEM, PAA Lab GmbH, E15-888) with 5.5 mM glucose, 2 mM stable glutamine and sodium bicarbonate, supplemented with 10% (v/v) fetal bovine serum (FBS) superior (Biochrom AG), 1% MEM nonessential amino acids (NEA, Biochrom AG) and 1% 4-(2-hydroxyethyl)piperazine-1-ethanesulfonic acid (HEPES, PAA Lab GmbH) at 37 °C with 5% CO 2 . The cells were split 2–3 times a week using trypsin/EDTA (Biochrom), supplemented with HEPES (PAA), sodium bicarbonate (PAA), penicillin/streptomycin (Biochrom) and PBS (Biochrom). The cells were transfected at 60–80% confluence with 5 μg DNA in 2.5 ml fresh medium. For the analysis of actively respiring mitochondria, the glucose medium was replaced with galactose medium (Dulbecco’s MEM=DMEM (PAA, E15-079)) with NEA, without glucose, and supplemented with 10 mM galactose (Sigma), 4 mM glutamine (Biochrom), 10% (v/v) fetal bovine serum (FBS) superior (Biochrom), sodium bicarbonate (PAA) and HEPES (PAA) for at least 2 days. For the analysis of hyperglycaemic mitochondria, the glucose medium was replaced by DMEM (PAA, E15-079), supplemented with 25 mM glucose (Sigma), 2 mM glutamine, 10% (v/v) fetal bovine serum (FBS) superior, sodium bicarbonate (PAA) and HEPES (PAA) for at least 2 days. For the protonophore and inhibitor studies, the cells were additionally treated with 10 μM CCCP (carbonyl cyanide m-chlorophenyl hydrazone, Enzo Life) for at least 30 min and 5 μg ml −1 oligomycin (Enzo Life, times indicated) or 3 mM KCN (potassium cyanide, Sigma) for 10–30 min. Ratio imaging microscopy for pH determination Two days after the transfection with sEcGFP fusion constructs, the pH of the transfected cells was recorded in situ by confocal fluorescence emission ratio imaging (inverted Olympus Fluoview FV1000). The cLSM was equipped with a × 60 oil immersion objective (UPLSAPO oil, NA 1.35, ∞/0.17/FN26.5) and two spectral detectors. All measurements were performed at room temperature in fresh growth medium. Ratio images were obtained simultaneously using the NIR laser (ex. 405 nm) of the microscope (em. 454–474 nm and 508–514 nm). In situ pH calibration For pH calibration, cells were perfused initially for 3–5 min with PBS (PAA, pH 7.0–7.5 with CaCl 2 and MgCl 2 ). Then, PBS was exchanged for MES (pH 5.6–6.1), BES (pH 6.1–7.6) or HEPPSO (pH 7.1–8.0) buffer, which was adjusted to the desired pH by 1 M HCl or NaOH, and supplemented with the following compounds: 125 mM KCl, 20 mM NaCl, 0.5 mM CaCl 2 , 0.5 mM MgSO 4 , 20 μM CCCP, 1 μM nigericin and 5 μg ml −1 oligomycin. Images were obtained within 15-45 min of incubation. Nigericin was purchased from Enzo Life. MES was purchased from Biomol, and BES and HEPPSO were purchased from Sigma. Other commonly used chemicals were purchased from Roth. Membrane potential measurements The membrane potential was determined with 5 nM TMRE and without quenching after 30 min of incubation with verapamil (10 μM) to block the multidrug transporter. In brief, verapamil and 5 nM TMRE were added to the incubation medium for 30 min at 37 °C. Then, the cells were mounted into a chamber with fresh incubation medium containing 5 nM TMRE and 10 μM verapamil for microscopy studies. Thus, measurements were performed using equilibrated dye. The fluorescence of mitochondrial TMRE in the mitochondrial regions of interest was then determined using the same settings (gain and fluorescence excitation power) in all samples. Because the cells were transiently transfected, an internal control was always available. Data were analysed by using ImageJ software (NIH Image, http://rsb.info.nih.gov/nihimage/index.html ). The mean grey values of mitochondrial TMRE (lines along site mitochondria ~3 μm, pixel size: 1 px=0.166 μm site) were determined. Because the uncoupling of mitochondria after the addition of CCCP (10 μM) led to an almost complete disappearance of the TMRE signal, we concluded that the measurements were performed without quenching. Data analysis The data were analysed by using ImageJ software (NIH Image, http://rsb.info.nih.gov/nihimage/index.html ) according to the procedure from Morgan et al . [37] In brief, to determine intracellular pH maps, background-subtracted images were processed using the sigma filter option of the ImageJ software (pixel radius=1, pixels used within 2 sigmas, minimum pixel fraction=0.4) and scaled up to 5. Then, a threshold level for the converted 32-bit images was determined interactively for each cell. The threshold was determined only for the images recorded at λ e =508–514 nm because these images had higher signal/noise ratios and were divided by the images with the lower signal/noise ratio. The background was set to NaN. For the final image, another threshold was set to >1, and the ratio was determined. All the background pixels were set to NaN in the images; within the cells, each pixel represents the ratio of the emission at 508–514 nm to that at 454–474 nm. The Boltzmann fit was chosen here for fitting the sigmoidal curves of the calibration data, in accordance with Grynkiewicz [38] , who described the relation between analyte concentration and fluorescence and fluorescence ratios. The fitting was performed using Origin 6.0 (OriginLab Corp., Northhampton, MA, USA). How to cite this article: Rieger, B. et al . Lateral pH gradient between OXPHOS complex IV and F 0 F 1 ATP-synthase in folded mitochondrial membranes. Nat. Commun. 5:3103 doi: 10.1038/ncomms4103 (2014).